Fathers are just as good as mothers at recognizing the cries of their baby Previous investigations of parents’ abilities to recognize the cries of their own babies have identified substantial and significant sex differences, with mothers showing greater correct recognition rates than fathers. Such sex differences in parenting abilities are common in non-human mammals and usually attributed to differential evolutionary pressures on male and female parental investment. However, in humans the traditional concept of ‘maternal instinct’ has received little empirical support and is incongruous given our evolutionary past as cooperative breeders. Here we use a controlled experimental design to show that both fathers and mothers can reliably and equally recognize their own baby from their cries, and that the only crucial factor affecting this ability is the amount of time spent by the parent with their own baby. These results highlight the importance of exposure and learning in the development of this ability, which may rely on shared auditory and cognitive abilities rather than sex-specific innate predispositions. The notion of maternal instinct has long been a topic of controversy [1] , [2] . Although it is now accepted that human behaviour emerges from complex interactions between genetics and environment [3] , [4] , [5] , [6] , the view that human mothers have better parenting skills than fathers, and that this sexual dimorphism has a strong genetic basis, is still widespread among the non-specialist public and biologists [7] , [8] , [9] . According to this view, women possess innate behavioural predispositions to assess their baby’s needs and to provide adapted care that men lack. In humans, crying is the main mean whereby newborns communicate their distress or needs and is equivalent to separation or begging calls uttered by youngsters of other mammals [10] , [11] . The ability to recognize their baby from their cries may contribute along with other cues to parents’ ability to identify their offspring among others (especially in the absence of visual cues). Moreover, the ability to familiarize themselves with the individual characteristics of their offspring’s cries is likely to facilitate caregivers’ assessment of intra-individual variation in cries (known to encode qualitative and quantitative information on condition, needs, emotional status and degree of urgency), thus enabling them to provide adapted care [12] . According to the ‘maternal instinct’ hypothesis, mothers should be better than fathers in performing these tasks. Although the very few experiments that have investigated individual recognition of human infant cries by parents mostly focused on mothers [13] , [14] , [15] , [16] , two studies that included parents of both sexes indeed reported that mothers performed much better than fathers [15] , [16] , giving support to the ‘maternal instinct’ hypothesis. However, because neither study controlled for the amount of time spent by parents of either sex with their baby, they failed to disentangle the possible effect of sex differences in exposure and learning from the possible effect of sex-specific genetic predisposition in the development of this ability. In recent years, the cooperative breeding hypothesis has challenged the view of ‘maternal instinct’ by suggesting that the human species is characterized by high levels of non-maternal care: fathers and other non-mother people directly provide care to babies [17] . Cross-cultural studies indeed show that paternal care is widespread in our species, making it a remarkable feature of human reproduction compared with what is observed in other mammals [18] , [19] . The cooperative breeding hypothesis implies that skills for offspring care are not restricted to mothers, hence limiting the relevance of maternal instinct. However, the psychological and cognitive correlates of the cooperative breeding model have not yet been systematically documented [20] and our understanding of differences in abilities to care for babies between mothers and non-mother caregivers remains insufficient [17] , [21] . The aim of the present study is to compare the ability of mothers and fathers to identify their baby among others from listening to their cries, while controlling for the amount of time spent by the parent with their baby. A better ability of mothers to perform this task compared with fathers would support the idea of a specialized female predisposition. Here we present the first controlled experimental evidence that both fathers and mothers reliably and equally recognize their own baby from their cries, emphasizing that recognition abilities result from an efficient learning process, independently of the parent’s sex. Individual differences in babies’ cries We analysed the cries of 29 babies (17 boys, nine from France and eight from Democratic Republic of Congo, and 12 girls, six from France and six from Democratic Republic of Congo; aged from 58 days to 153 days, median=115 days). Sampling babies from two different countries increased the diversity of parental contexts, for example, the amount of time spent by each parent with their baby and their concurrent exposure to other babies (nuclear versus enlarged families). Spontaneous cries were recorded on three different days, during the same bathing context. Two 8 s sequences of crying were isolated from each recording event, resulting in six sequences per baby. To assess the individual signature, we characterized the cries’ acoustic structure using a set of temporal and spectral parameters and used these parameters in cross-validated and permuted discriminant function analyses (DFA). Infant cries were individually different: the classification success rate across individuals was significantly greater than chance (mean of correct classification=33.5±17.8%, chance=3.4%, P <0.001 using permuted DFA, Fig. 1a , Supplementary Audio 1–4 ). 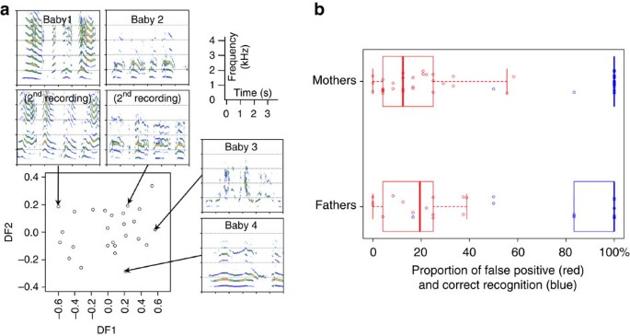Figure 1: Individual identification of human babies’ cries. (a) Analysis of the individual signature in cries: each point in the central graph represents the centroid of a baby’s cries as a function of the first two discriminant variables that maximize individual separation. The mean fundamental frequency and the maximal value of the fundamental frequency are the two main factors that separate individuals on the first function (DF1,Table 1). The second function (DF2,Table 1) relies mostly on the maximal value of the fundamental and the periodic quality of the signal (parameter ‘jitter’, see Methods section). Spectrograms on the sides illustrate the differences in acoustic structure between cries of different babies. Two cries coming from two different recording sessions are illustrated for the babies 1 and 2, showing the individual consistency of individual cries (to hear the sounds:Supplementary Audio 1–4corresponding to babies 1–4). (b) Playback experiments testing parental recognition of their baby’s cry: correct recognition (in blue) and false positive (in red) by parents spending at least 4 h a day with their baby. Circles represent the values for each of the tested parents (N=29 mothers and 14 fathers). Box and whisker plots report the median, 25th and 75th percentiles, and the lowest and highest data, which are no more than 1.5 × interquartile range from the box. Both fathers and mothers reliably identify their babies on the basis of cries only. Differences between fathers and mothers are not statistically significant (see main text andTables 3,4,5for statistics). Table 1 reports the relative weight of acoustic parameters on the first three discriminant functions, emphasizing the importance of fundamental frequency and its modulation. Table 2 reports the mean values of all measured acoustic variables. Figure 1: Individual identification of human babies’ cries. ( a ) Analysis of the individual signature in cries: each point in the central graph represents the centroid of a baby’s cries as a function of the first two discriminant variables that maximize individual separation. The mean fundamental frequency and the maximal value of the fundamental frequency are the two main factors that separate individuals on the first function (DF1, Table 1 ). The second function (DF2, Table 1 ) relies mostly on the maximal value of the fundamental and the periodic quality of the signal (parameter ‘jitter’, see Methods section). Spectrograms on the sides illustrate the differences in acoustic structure between cries of different babies. Two cries coming from two different recording sessions are illustrated for the babies 1 and 2, showing the individual consistency of individual cries (to hear the sounds: Supplementary Audio 1–4 corresponding to babies 1–4). ( b ) Playback experiments testing parental recognition of their baby’s cry: correct recognition (in blue) and false positive (in red) by parents spending at least 4 h a day with their baby. Circles represent the values for each of the tested parents ( N =29 mothers and 14 fathers). Box and whisker plots report the median, 25th and 75th percentiles, and the lowest and highest data, which are no more than 1.5 × interquartile range from the box. Both fathers and mothers reliably identify their babies on the basis of cries only. Differences between fathers and mothers are not statistically significant (see main text and Tables 3 , 4 , 5 for statistics). Full size image Table 1 Acoustic parameters’ loading on the first three discriminant functions. Full size table Table 2 Acoustic characteristics of babies’ cries. Full size table Recognition by parents We assessed parents’ ability to recognize their own baby on the basis of their cries, against the cries of other same-aged babies (number of parents tested: 27 fathers and 29 mothers). Each parent was tested with a playback trial including two sessions of 15 cries (each session included three different cries from five babies with cries from the infant of the parent tested, two unknown boys and two unknown girls of similar age; cries were presented in randomized order). The experimenter was blind to the conditions, and participants knew neither how many cries were from their own child, nor how many different babies they originated from. On average, parents identified 5.4±1.2 out of the six cries of their baby (mean recognition rate=90±21%). The number of false-positive errors was 4.1±3.2 among 24 possible (mean rate of false positive=17±14%). The time spent with the baby and the exposure to other babies were important factors in determining parental response. Thus, for a similar time spent with their infant (>4 h per day), fathers succeed as well as mothers ( Fig. 1b ; mean recognition rate=90±9% for fathers, N =14, and 98±10% for mothers, N =29, χ 2 =0.47, P =0.49 using a linear mixed-effect model (LME); mean rate of false positive=20±14% for fathers and 16±15% for mothers, χ 2 =0.23, P =0.63 using a LME; Table 3 ). Among fathers, those who spent less than 4 h per day with their infants ( N =13) had a significantly lower rate of recognition (75±28%, χ 2 =5.3, P =0.02 using a LME; Table 4 ). Parents who were daily exposed to other babies ( N =20) had a lower recognition rate (82±30%, χ 2 =9.50, P =0.02 using a LME; Table 5 ) and a higher rate of false positive (25±15%, χ 2 =8.308, P <0.01 using a LME; Table 5 ) than those who were only exposed to their own infant cries (recognition rate=95±12%, false positive=14±12%, N =36). Interaction between parental sex and exposure to other babies was not significant ( Table 5 ). Babies’ sex, babies’ age and the number of children previously raised affected neither the rate of recognition nor the rate of false positives ( Table 5 ). The significant effects of number of previously raised children and its interaction with time spent with baby reported in Table 4 should be treated cautiously. Indeed, most of the fathers ( N =25) in our sample had between one and four children, whereas very few ( N =2) had more than four. Besides, there was a significant effect of the interaction between baby sex and time spent. However, given the small sample size (five fathers having daughters versus eight having sons), this effect requires further investigation before solid conclusions can be drawn. Finally, in the model reported in Table 5 , parent sex and time spent are non-independent factors as, in our sample, no mother spent less than 4 h a day with their baby: the effect of the interaction between infant age and parent sex and the effect of the interaction between infant sex and time spent are better examined using the more suitable models reported in Table 3 (based on parents spending more than 4 h per day with their infant) and in Table 4 (based on fathers only). Table 3 Summary of LMEs from parents spending more than 4 h per day with their infant. Full size table Table 4 Summary of LMEs from the fathers only. Full size table Table 5 Summary of LMEs from both fathers and mothers. Full size table Studies of infant vocal recognition abilities in human parents conducted in the late seventies and early eighties reported that mothers performed well, and better than fathers when completing this task (recognition rates of 97 versus 84%, with false-positive rates of 25 and 56% (ref. 15 ); recognition rates of 80 versus 45% (ref. 16 )). These results were in line with popular beliefs that are still prevailing today, as exposed by the results of a survey that we recently performed on 531 participants from University de Saint-Etienne (all naive to the present study): while 43% of the questioned participants thought that mothers were better than fathers at recognizing their baby, none thought that the reverse was true (unpublished results). Conversely, the results presented here clearly show that fathers and mothers are equally highly successful at identifying their babies from listening to their cries, and that the amount of time spent by participants with their baby appears to be the main factor affecting this ability. The difference between our results and those of previous studies may therefore derive from the fact that they did not control for variation in time spent by participants with their own baby. Our study therefore suggests an important role of experience, rather than sex-specific innate predispositions, in determining a parent’s ability to recognize their own baby from their cries. Indeed, women do not appear to have evolved specialized skills, and parents of both sexes may rather make use of shared auditory and cognitive abilities. Further studies should however investigate more precisely the effect of time spent (measured as a continuous variable) with own baby on recognition skills in both mothers and fathers. That would allow us to establish how a wider range of exposure affects recognition skills, and whether it similarly affects parents of both sexes. We also found that daily contact with others’ babies impaired the ability of parents to recognize their own baby, indicating that exposure to the cries of different babies may affect parents’ ability to learn the vocal signature of their own child. We suggest that the increase in false-positive responses to other babies’ cries associated with these parents could represent a strategy aimed at decreasing the risk of not responding to their own baby. Endocrinological studies have shown that hormonal levels can be correlated with parental behaviour [22] , [23] . For example, testosterone levels decrease in men when they become fathers [22] . Future investigations could therefore examine the relationship between hormonal state and baby recognition in fathers by, for example, testing whether testosterone levels and time spent with baby correlate, and whether testosterone levels influence recognition abilities. Mothers and fathers are likely to develop comparable recognition abilities in species where both parents provide parental care. This includes all monogamous species. In addition, our observations are likely to also be consistent with the currently accepted view that humans were cooperative breeders during a long part of their evolutionary history [20] . Individual recognition from cries is thus likely to have supported the process of psychological attachment by any caregiver—mother, father and others. Yet, the abilities of non-parent caregivers would still have to be tested to fully support this argument. Parental recognition abilities may not be a sex-specific adaptation supporting the restriction of care to the mothers’ own infant, but rather a general ability shared by both parents and mainly affected by experience. Subjects The study was carried out on 29 families. Fifteen families were located in Saint-Etienne, France, and 14 families lived in two villages in Democratic Republic of Congo. The research was performed under the authorization no. 42-218-0901 SV09 (ENES Lab, DDSVL) and approved by the local CNIL committee. Informed consent was obtained from all subjects. Questionnaire Each parent answered a questionnaire during an individual interview. Information was gathered on the number of children raised. Information was also gathered on the time spent with the infant per day (excluding time when the baby is asleep). All mothers spent more than 4 h per day with their baby. Fathers could be divided into two categories: those who spent more than 4 h per day with their infant (median=5.5, Q 1–3 =4.5–8, N =14) and those who spent less than 4 h per day with their infant (median=3, Q 1–3 =2–3, N =13). Two categories of families were distinguished regarding to the exposure to other babies’ cries. One category was the ‘nuclear family’, whereby the parent was mostly exposed only to the cries of their own baby, and only occasionally heard the cries from other babies (less than once per week); N =36 parents (17 men, 19 women). The other category was the ‘enlarged family’, whereby the parent was exposed to the cries of other babies (<1 year old) on a daily basis; N =20 parents (10 men, 10 women). All mothers from enlarged families, and 16 out of the 19 mothers from nuclear families breast-fed their child during at least 2 months after birth. Sound recordings All cries were collected during the context of bathing, that is, during undressing, bathing and dressing when babies expressed their unhappiness at being manipulated or put into water. All recordings came from spontaneous cries. If the infant did not cry, we attended a new bath another day. In total, each infant was recorded at three independent bath events. Recordings were performed with a microphone (Sennheiser MD42), placed at 30 cm from the baby and connected to a recorder (Marantz PMD690/W1B in France, and Edirol in DRC). To limit pseudo replication we isolated two sequences of crying of around 8 s each (mean±s.d.=8.2±1.1) from each bath event using Avisoft software (Avisoft-SASLab Pro Version 4.39) resulting in a total of six sequences for each baby. Sound analyses We performed acoustic analyses using a dedicated batch-processing script in PRAAT [24] , which contained four distinct procedures. The first procedure of the script characterized the fundamental frequency (F0) and the intonation (F0 contour variation) of the cries. The F0 contour was extracted using the To Pitch (cc)… , command. The experimenter systematically inspected the extracted Pitch contour and verified it using a narrow band spectrogram displaying the first 2,000 Hz of the signal. Spurious octave jumps were manually corrected by selecting the appropriate F0 candidate values in the edited pitch object. In the relatively rare segments including double vibration (where a weak subharmonic equal to half the fundamental frequency is present), the F0 was systematically preferred over the subharmonic. Each extracted F0 contour (pitch object) was saved as a text file for future reference. These numerical representations were used to derive the following parameters: %voiced (percentage of the signal that is characterized by a detectable pitch), mean F0, max F0, min F0 (respectively the mean, maximum and minimum F0 calculated over the duration of the signal) and F0CV (coefficient of variation of F0 over the duration of the signal). In a second step, two distinct smoothing algorithms ( Smooth… command in Praat) were performed on the pitch contour: the first allowed a relatively broad bandwidth ( Smooth… command parameter=25), to suppress very short-term frequency fluctuation while preserving minor intonation events (such as bleat-like frequency modulation), and the second only allowed a narrow bandwidth ( Smooth … command parameter=2), to only characterize strong F0 modulation (major intonation events). Inflection points were counted (as each change in the sign of the contour’s derivative) after each smoothing procedure, and divided by the total duration of the voiced segments in each recording, resulting in two distinct indexes of F0 variation (inflex25 and inflex2). A second procedure focused on the intensity contour and allowed the characterization of the variability of the cries’ intensity by calculating intCV, the coefficient of variation of the intensity contour estimated using the To intensity … command in PRAAT. A third procedure focused on the periodic quality of the signal and measured the harmonicity (harm, degree of acoustic periodicity, measured as the ratio of harmonics to noise in the signal and expressed in dB), an index of jitter (jitter, small fluctuation in periodicity measured as the average of ‘local’, ‘rap’ and ‘ppq5’ measures in PRAAT [24] ) and an index of shimmer (shimmer, small variation in amplitude between consecutive periods, measured as the average of ‘local’, ‘apq5’ and ‘apq11’ parameters in PRAAT [24] ). A final procedure characterized the spectral envelope of the cry by applying a cepstral smoothing procedure (bandwidth: 900 Hz) to each crying sequence, followed by the extraction of the first four spectral prominences (SP1, SP2, SP3, SP4) of the resulting smoothed spectrum. Because babies’ cries can be strongly nasalized [25] , and can contain biphonation phenomena (Soltis [10] , our observation) that can create resonance-independent broadband components, the measured spectral peaks cannot be safely considered as accurate measure of formant frequencies and are therefore termed spectral prominences. However, the observed values 1.2, 3.1, 5.7 and 8.6 kHz are consistent with the newborn/infant vocal tract length ( ∼ 7.5 cm between 2 and 6 months [26] predicting vocal tract resonances are at about 1.1, 3.3, 5.5 and 7.7 kHz). Statistical analysis of individual signatures We used a cross-validated and permuted DFA [27] . A fitting data set (2/3 of the sounds from each individual) was used to generate linear discriminant functions on the basis of the 15 measured acoustic features described above. The remaining 1/3 of the sounds were used as a cross-validation set to measure the effect size (the percentage of correctly classified sounds) using the discriminant functions obtained with the fitting set. The mean effect size was calculated from 100 random iterations. To obtain the statistical significance of the effect size, data sets where the identity of sounds was randomly permuted between individuals were created (permuted DFA). The same steps, fitting and validating, were followed for each of these randomized sets. After 1,000 iterations, the proportion of the randomized validation data sets revealing the number of correctly classified sounds as large as the effect size obtained with the non-randomized validation data set was calculated. This proportion gives the significance of the discrimination level and is equivalent to a P -value [28] . Playback experiments A playback test included two sessions of 15 cries separated by few minutes. Each session contained three different cries from five distinct babies including cries from the infant of the parent tested, two boys and two girls. The cohort in playback sessions was chosen to have similar age (less than 20 days of difference). All the cries were randomized. Both parents of a given infant listened to the same five baby identities but randomized differently. For four infants out of 29, only four or five sequences of cries could be isolated from the three bath events. In these cases, a same cry had been used twice but in a different playback session. During a playback experiment, the subject listened to 30 cries through Sennheiser HD 25–1 headphones. The delay between the playback test and the latest recording was 6±8.6 days. To avoid potential influence of the experimenter, the playback test was conducted as a double-blind experiment. Tracks were encoded and the adult tested knew neither how many cries originated from their child nor how many different babies were broadcasted. For each cry, we asked the parent if it was his/her infant or not. Analysis of parental responses The responses of adults were expressed as a binary answer (wrong/correct) for each cry. We used LME models with binomial distribution to examine the effects of the infant’s age and sex, the number of children raised by the parent tested, the exposure to other babies’ cries, the parent sex and the time spent with the baby on the rate of recognition and the rate of false positive. Individual identity of the parent tested was included as a random effect in LMEs as each parent responded repeatedly (that is, for the 30 cries). Initially, all explanatory variables and the two-way interactions were fitted in a maximal model. Then, nonsignificant interactions and main terms were dropped sequentially to simplify the model. All the mothers tested spent more than 4 h per day with their infant so we did not test the interactions ‘parent sex × time’. Additional LMEs were fitted to compare between mothers and fathers within the parents spending more than 4 h per day with their infant and to test the effect of the time spent with the baby within the fathers. All LMEs were fitted using R (v. 2.14.1; R Development Core Team 2011). How to cite this article: Gustafsson, E. et al . Fathers are just as good as mothers at recognizing the cries of their baby. Nat. Commun. 4:1698 doi: 10.1038/ncomms2713 (2013).